Ir-catalyzed enantioselective B−H alkenylation for asymmetric synthesis of chiral-at-cageo‑carboranes The asymmetric synthesis of chiral-at-cage o -carboranes, whose chirality is associated with the substitution patterns on the polyhedron, is of great interest as the icosahedral carboranes have wide applications in medicinal and materials chemistry. Herein we report an intermolecular Ir-catalyzed enantioselective B−H alkenylation for efficient and facile synthesis of chiral-at-cage o -carboranes with new skeletons under mild reaction conditions. Generally very good to excellent yields with up to 99% ee can be achieved in this Ir-catalyzed B−H alkenylation. The enantiocontrol model is proposed based on Density Functional Theory calculations in which the use of chiral phosphoramidite ligand is essential for such asymmetric o -carborane B−H alkenylation. Stereochemistry has been one of the most active research areas in modern chemistry. Asymmetric catalysis with chiral metal complexes, enzymes, and chiral organic molecules have emerged as successful and powerful tools in asymmetric synthesis to obtain enantiomerically enriched compounds [1] , [2] , [3] , [4] , [5] . Despite a great variety of chiral structures incorporating central, axial, planar, and helical chirality achieved by catalytic asymmetric synthesis, to obtain the inherent chirality of three-dimensional cage compounds such as carboranes is extremely challenging and the currently available methods to access such an enantioenriched skeleton are still rather limited [6] , [7] , [8] , [9] . Icosahedral carboranes are carbon–boron molecular clusters, often viewed as three-dimensional analogs to benzene, which are invaluable building blocks for applications ranging from functional materials to pharmaceuticals [10] , [11] , [12] , [13] , [14] , [15] , [16] , [17] , [18] . The most extensively studied o -carborane, which shows a highly symmetrical 3D structure and extraordinary versatility [19] , [20] , [21] , [22] , can be transformed to chiral-at-cage molecules with the addition of substituents to lower the symmetry of its icosahedral structure [23] , [24] , [25] , [26] , [27] . In view of the rapidly developed transition-metal-catalyzed regioselective o -carborane B–H bond activation methodologies [28] , [29] , [30] , [31] , [32] , [33] , [34] , controlled introduction of a substituent at either cage B(4) or B(5) of C(1)-substituted o -carboranes would be possible, resulting in the chirality of the resultant molecules (Fig. 1 ) [35] . Inspired by the recent reports on fullerene cage chirality [36] , [37] , [38] , [39] and ferrocene planar chirality [40] , the transition-metal-catalyzed enantioselective B–H functionalization should realize the synthesis of optically pure chiral-at-cage o -carborane derivatives, which are important in the fields of asymmetric synthesis, materials science, and medicinal chemistry, where the chirality plays an important role in molecular design. We have very recently reported a proof-of-concept study on enantioselective synthesis of chiral-at-cage o -carborane derivatives via a Pd-catalyzed intramolecular B(5)–H arylation of o -carboranes in the presence of chiral phosphine ligands [41] . Fig. 1: The inherent cage B(4/5) chirality of 1,2-substituted- o -carboranes. The presence of a substituent at the position 4/5 results in the chirality of the molecule. The observer looks onto the pentagonal plane of C(2)–B(3)–B(4)–B(5)–B(6) in o -carborane and then examines the position of the substituent according to the Cahn–Ingold–Prelog rule for the determination of the cage chirality. Full size image Herein, we report an intermolecular catalytic asymmetric B−H functionalization of o -carboranes with the assistance of a directing group and chiral phosphoramidite ligand. This protocol allows easy access to chiral-at-cage o -carborane derivatives in high yields and excellent enantioselectivities via Ir-catalyzed enantioselective B−H alkenylation under mild reaction conditions. It illustrates an important application of asymmetric synthesis beyond conventional organic chemistry into the chemistry of chiral boron cages. Reaction development and optimization We initially examined the regioselectivity of the reaction using 1-acetylamino-2-methyl- o -carborane ( 1a ) and diphenylacetylene ( 2a ) as model coupling partners and [Cp*IrCl 2 ] 2 as a precatalyst. 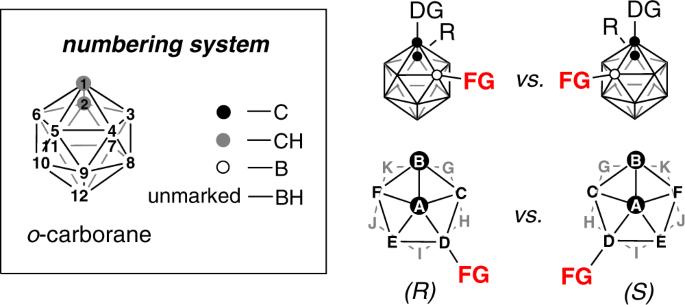Fig. 1: The inherent cage B(4/5) chirality of 1,2-substituted-o-carboranes. The presence of a substituent at the position 4/5 results in the chirality of the molecule. The observer looks onto the pentagonal plane of C(2)–B(3)–B(4)–B(5)–B(6) ino-carborane and then examines the position of the substituent according to the Cahn–Ingold–Prelog rule for the determination of the cage chirality. Reaction of 1a with 2 equiv of 2a in toluene at 80 °C in the presence of 5 mol% [Cp*IrCl 2 ] 2 , 25 mol% AgNTf 2 , 2 equiv of Cu(OAc) 2 , and 5 equiv of PhCO 2 H afforded the desired B(4/5)-alkenylation product 3aa as a racemate in 83% isolated yield with complete regioselectivity (B(4/5) vs. B(3/6)) (Table 1 , entry 1). Two enantiomers were able to be separated by HPLC on the Chiralpak IA column (see Supplementary Fig. 283 ). To evaluate the feasibility of asymmetric B−H alkenylation, we then evaluated the role of chiral ligands, and the results were compiled in Table 1 . Bisphosphine ligand ( S )-BINAP L1 deactivated the catalyst, whereas monophosphine ligand ( R )-MOP L2 and ( S )-BI-DIME L3 accelerated the alkenylation to yield 3aa quantitatively (Table 1 , entries 2–4) with no enantioselectivity. Among a series of chiral phosphoramidite ligands L4 – L14 examined, reactions with dibenz[b,f]azepine containing L8 – L14 provided promising results (Table 1 , entries 5–15). L8 , introduced by the Carreira group [42] , proved to be the most efficient chiral ligand in terms of enantioselectivity and reactivity, giving ( S )- 3aa in 72% isolated yield with 80% ee (Table 1 , entry 9). The use of a stronger acid, phenylsulfonic acid, as an additive, improved the reaction efficiency (Table 1 , entry 16). It was later found that the cage C-benzylated substrate, 1-acetylamino-2-benzyl- o -carborane ( 1b ), significantly enhanced the enantioselectivity to 93% ee (Table 1 , entry 17). Table 1 Screening of chiral ligands and additives a . 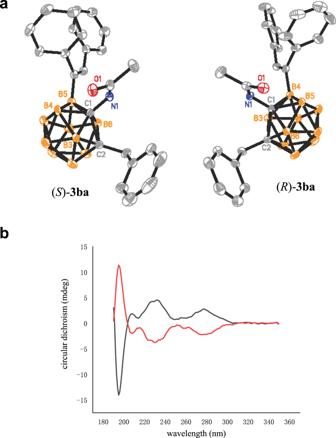Fig. 2: The chirality of B(4/5)-alkenylatedo-carborane. aMolecular structures of (S)-3baand (R)-3ba.bCD Spectra of (S)-3ba(black) and (R)-3ba(red) in MeCN (c= 0.1 mg/mL). Full size table After a systematic evaluation of reaction parameters such as solvents, acids, [Ag], and [Cu] additives (see Supplementary Tables 1 – 3 for detail), the asymmetric intermolecular alkenylation of 1b proceeded smoothly in toluene under the “normal” conditions (Table 2 , entry 1), giving ( S )- 3ba in 99% yield and 94% ee. Further screening of the catalysts indicated that Pd(OAc) 2 provided the product in high yield with poor enantioselectivity, whereas [Cp*RhCl 2 ] 2 and IrCl 3 showed no catalytic activity (Table 2 , entries 2–4). To our surprise, improved enantioselectivity of 97% ee was observed with [Ir(COD)Cl] 2 as an Ir precursor in the absence of Cu(OAc) 2 (Table 2 , entries 5–6). Lowering the reaction temperature to 50 °C resulted in an increased ee to 99% (Table 2 , entry 7). The 2.5 mol% catalyst loading also worked very well (Table 2 , entry 9). It was noted that a complete reversal of the enantioselectivity was observed with ( R )- L8 ligand (Table 2 , entry 10). Table 2 Optimization of Ir-catalyzed asymmetric B–H alkenylation a . Full size table The circular dichroism (CD) spectra of ( R )- 3ba and ( S )- 3ba exhibited unambiguously mirror images to each other, indicating a pair of enantiomers. The absolute configurations of ( R )- 3ba and ( S )- 3ba were determined via single-crystal X-ray analyses (Fig. 2 ). In addition, the single-crystal X-ray structure and CD spectrum of ( S )- 3bd (see the Supplementary Information for detail) further confirm the assignment of the absolute configurations for ( R )- 3ba and ( S )- 3ba . Fig. 2: The chirality of B(4/5)-alkenylated o -carborane. a Molecular structures of ( S )- 3ba and ( R )- 3ba . b CD Spectra of ( S )- 3ba (black) and ( R )- 3ba (red) in MeCN ( c = 0.1 mg/mL). Full size image Substrate scope Under the optimized reaction conditions (Table 2 , entry 9), the alkyne substrate scope was then examined and the results were summarized in Fig. 3 . Generally, diaryl acetylenes with electron-withdrawing groups such as –F, –Cl, –Br, –CF 3, and –CO 2 Me worked very well, affording ( S )- 3bb – 3bf , 3bm, and 3bq in excellent yields with 89–99% ee. p -Acyl and p -phenyl were also tolerated with low conversions and enantioselectivities ( 3bg , 3bh ). For the electron-donating group containing substrates, a higher reaction temperature of 80 °C was required to promote the reaction, leading to slightly decreased enantioselectivity. It was found that the addition of 1.1 equiv of Cu(OAc) 2 to the above reactions could not only accelerate the reaction but also improve the enantioselectivity ( 3bi – 3bk , 3bn – 3bp , 3br , 3bs ) with a lower reaction temperature probably due to the activation of alkynes via their complexation with Cu(II) salt. Steric factors also played a role as di- o -tolylacetylene was not compatible. Unsymmetrical alkyne MeC≡CPh gave two regioisomers of 3bt and 3bt ′ in a 4:1 ratio with 58% and 60% ee, respectively. Fig. 3: Alkyne substrates scope and molecular structures of ( S )-3bd and ( S )-3bs. General conditions: 1b (0.1 mmol), 2 (0.12 mmol), 2.5 mol% [Ir(COD)Cl] 2 , 5 mol% ( S )- L8 , 12.5 mol% AgNTf 2 , 1.5 equiv of C 6 H 5 SO 3 H in 2 mL of toluene, 50 °C, 40 h. [Ir(COD)Cl] 2 and ( S )- L8 was dissolved in 1 mL of toluene and stirred at r.t. for 1 h in advance; isolated yields. ee enantiomeric excess. a 12 h. b 4 days. c 80 °C. d 1.1 eq. of Cu(OAc) 2 was added. e The ratio was determined by 1 H NMR. Full size image For the scope of o -carboranes (Fig. 4 ), cage C substituent R 1 does not have an obvious impact on the reactions except for R 1 = H ( 3ca ), affording the corresponding ( S )-B(5)-alkenylated compounds ( 3aa , 3ba , 3da – 3ha ) in high yields (94−99%) with excellent enantioselectivity (92−99% ee). For B(9,12)-dimethylated o -carborane, a lower alkenylation efficiency was observed, but the enantioselectivity remained unchanged ( 3ia ; 60% yield, 99% ee). On the other hand, bulky substituent R 3 on the amide group resulted in slightly low yields and enantioselectivities ( 3na – 3ra ). Fig. 4: o -Carborane substrates scope and molecular structure of ( S )-3ha. General conditions: 1 (0.1 mmol), 2 (0.12 mmol), 2.5 mol% [Ir(COD)Cl] 2 , 5 mol% ( S )- L8 , 12.5 mol% AgNTf 2 , 1.5 equiv of C 6 H 5 SO 3 H in 2 mL of toluene, 50 °C, 40 h. [Ir(COD)Cl] 2 and ( S )- L8 was dissolved in 1 mL of toluene and stirred at r.t. for 1 h in advance; isolated yields. ee enantiomeric excess. a 12 h. b 80 °C. c 4 days. d 1 week. Full size image A large-scale synthesis of ( S )- 3ba was subsequently carried out (Fig. 5a ). Under the optimal reaction conditions, treatment of 1b (582 mg, 2.0 mmol) with 1.2 equiv of diphenylacetylene (428 mg, 2.4 mmol) in the presence of 2.5 mol% [Ir(COD)Cl] 2 , 5 mol% ( S )- L8 , 12.5 mol% AgNTf 2 and 1.5 equiv of C 6 H 5 SO 3 H in toluene (20 mL) afforded ( S )- 3ba (860 mg, 92% isolated yield) with 95% ee. In addition, the product ( S )- 3ba (98% ee) was readily converted to synthetically valuable amine by treatment with K 2 CO 3 in methanol, furnishing ( S )-1-NH 2 -2-Bn-5-[C(Ph)=CH(Ph)]- o -C 2 B 10 H 9 (( S )- 4ba ) in 90% yield with 97% ee (Fig. 5b ). Fig. 5: Large-scale synthesis of ( S )-3ba and its transformation. a Large-scale synthesis of ( S )- 3ba . b Deacylation of ( S )- 3ba . Full size image Compounds 3 and 4 were fully characterized by 1 H-, 13 C- and 11 B-NMR spectroscopy, as well as high-resolution mass spectrometry. The molecular structures of 3bd , 3bs, and 3ha were further confirmed by single-crystal X-ray analyses. Mechanistic investigations To gain some insight into the reaction mechanism, several control experiments were conducted. Under standard reactions, using C 6 H 5 SO 3 D as the acid additive gave ( S )- 3ba - d 1 in 98% yield and 99% ee with 20% D-incorporation (Fig. 6a ). On the other hand, treatment of 1b - d 8 with C 6 H 5 SO 3 H resulted in a 55% D-incorporation, suggesting some D–H exchange with the acid (Fig. 6b ). In the absence of C 6 H 5 SO 3 H additive, ( S )- 3ba - d 8 with >95% D-incorporation was obtained, indicating that the deuterium was originated from B(5)-D, and no deuterium scrambling over carborane was observed (Fig. 6c ). To gain additional information regarding the initial rate of the reaction, parallel reactions using substrate 1b and 1b - d 8 were conducted, leading to the kinetic isotope effect of k H / k D = 0.95 (Fig. 6d ; see Supplementary Figs. 11 and 12 for detail), which indicates that B−H activation is not involved in the rate-determining step. Fig. 6: Mechanistic investigations. Control experiments. a Reaction of 1b using C 6 H 5 SO 3 D as the acid additive. b Reaction of 1b - d 8 using C 6 H 5 SO 3 H as the acid additive. c Reaction of 1b without acid additive. d Independent-rate KIE experiments. Full size image As the Ir(I) can be oxidized by Ag(I) to generate in-situ active catalyst Ir(III) [43] that performs even better than [Cp*IrCl 2 ] 2 (Table 2 ), a plausible reaction mechanism is proposed in Fig. 7 . The catalysis is initiated by the Ir(III) generated in situ via the oxidation of [Ir(COD)Cl] 2 with Ag + in the presence of chiral phosphoramidite ligand, followed by the coordination with acetylamino- o -carborane 1 in an iminium form to offer the Ir(III) intermediate B . Subsequent selective electrophilic B(5)–H metalation [32] , [44] (for C–H metalation, see ref. [44] ) and alkyne insertion afford the intermediate D that undergoes protonation to give the final product 3 . Fig. 7: Proposed catalytic cycle. Possible reaction mechanism of the Ir-catalyzed enantioselective B−H alkenylation. The chiral ligand on Ir has been marked as L* for clarity. Full size image In the reaction, cage B(4/5) regioselectivity is dominated by the combination of the Ir(III) catalyst and the directing group [31] , [33] , whereas the enantioselectivity is controlled by the chiral phosphoramidite ligand [40] . ( S )- or ( R )- L8 leads to ( S )- or ( R )-enantiomer, respectively. To shed some light on the enantioselectivity in the current asymmetric B−H functionalization, the transition states TS- R and TS- S leading to the final alkenylation products in R and S configuration, respectively, were located by DFT calculations on the basis of concerted metalation-deprotonation (CMD) mechanism (Fig. 8 ). The B−Ir bond-forming step (from the intermediates B to C ) was identified as the stereoselectivity-determining step, leading to the preferentially generated ( S )-B(5)-alkenylation product. The transition state TS- S was calculated to be more stable than its enantiomer TS- R by 4.1 kcal/mol. Non-covalent interactions (NCI) analysis, which has been successful to identify electrostatic interactions, was performed using Multiwfn software [45] , [46] to gain further insight into the key factors that control stereoselectivity. The NCI pictures show that the π···π interactions exist in both isomers with nearly equal contributions (Fig. 8b ). The C-H···π interactions only exist in TS- S . These additional interactions would be responsible for stabilizing the transition state TS- S . Fig. 8: DFT calculated transition states. 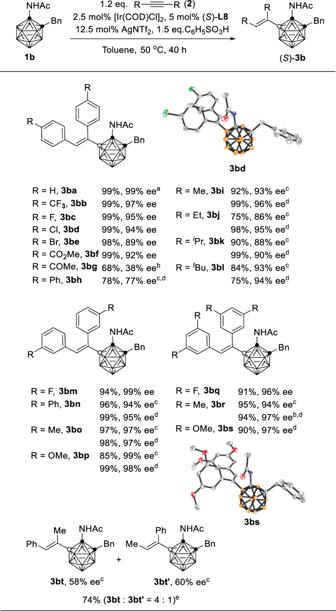Fig. 3: Alkyne substrates scope and molecular structures of (S)-3bd and (S)-3bs. General conditions:1b(0.1 mmol),2(0.12 mmol), 2.5 mol% [Ir(COD)Cl]2, 5 mol% (S)-L8, 12.5 mol% AgNTf2, 1.5 equiv of C6H5SO3H in 2 mL of toluene, 50 °C, 40 h. [Ir(COD)Cl]2and (S)-L8was dissolved in 1 mL of toluene and stirred at r.t. for 1 h in advance; isolated yields. ee enantiomeric excess.a12 h.b4 days.c80 °C.d1.1 eq. of Cu(OAc)2was added.eThe ratio was determined by1H NMR. a Structures of the two transition states TS- R and TS- S from the intermediates B to C . b NCI analysis for the enantioselective transition states TS- R and TS- S . Values in parentheses are distances between two interactive fragments in Å. Full size image In summary, the first intermolecular asymmetric B−H functionalization has been developed via Ir catalysis for the enantioselective synthesis of chiral-at-cage o -carboranes under mild reaction conditions. Generally very good to excellent yields with up to 99% ee can be achieved in this Ir-catalyzed B−H alkenylation. The enantiocontrol model is proposed based on DFT calculations in which the use of chiral phosphoramidite ligand is essential for such asymmetric o -carborane B−H functionalization. This work sets a good example for exploring the potential of asymmetric synthesis beyond conventional organic chemistry into the chemistry of chiral-at-cage o -carboranes. 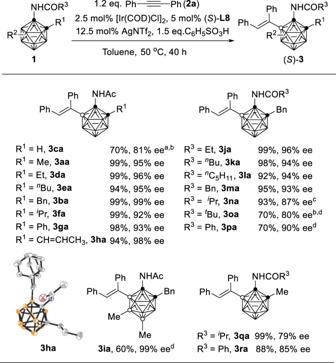Fig. 4:o-Carborane substrates scope and molecular structure of (S)-3ha. General conditions:1(0.1 mmol),2(0.12 mmol), 2.5 mol% [Ir(COD)Cl]2, 5 mol% (S)-L8, 12.5 mol% AgNTf2, 1.5 equiv of C6H5SO3H in 2 mL of toluene, 50 °C, 40 h. [Ir(COD)Cl]2and (S)-L8was dissolved in 1 mL of toluene and stirred at r.t. for 1 h in advance; isolated yields. ee enantiomeric excess.a12 h.b80 °C.c4 days.d1 week. 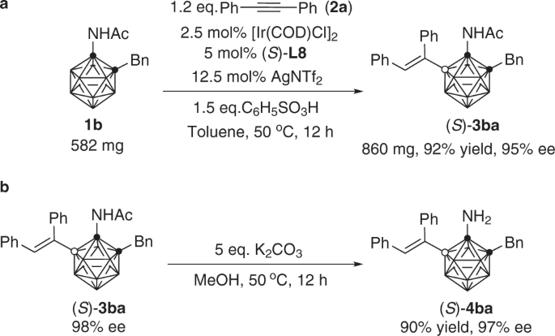Fig. 5: Large-scale synthesis of (S)-3ba and its transformation. aLarge-scale synthesis of (S)-3ba.bDeacylation of (S)-3ba. A representative procedure for the synthesis of 3 An oven-dried Schlenk flask equipped with a stir bar was charged with [Ir(cod)Cl] 2 (1.7 mg, 0. 0025 mmol) and ( S )- L8 (2.6 mg, 0.005 mmol), followed by dry toluene (1 mL). The mixture was stirred at room temperature for 1 h, to which was successively added 1 (0.10 mmol), 2 (0.12 mmol), benzenesulfonic acid (24 mg, 0.15 mmol), AgNTf 2 (4.9 mg, 0.0125 mmol), and dry toluene (1 mL). The flask was closed under an atmosphere of nitrogen, then stirred at 50 °C for 40 h. After hydrolysis with water (5 mL) and extraction with diethyl ether (10 mL × 3), the ether solutions were combined, dried over anhydrous Na 2 SO 4, and concentrated to dryness in vacuo. The residue was subjected to flash column chromatography on silica gel (230–400 mesh) using n -hexane and ethyl acetate (4/1 in v/v) as eluent to give the product ( S )- 3 . 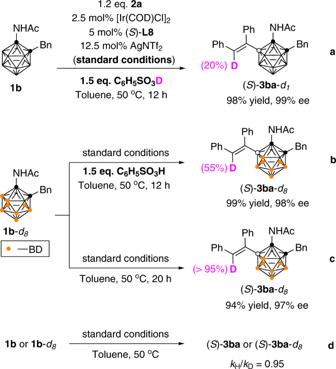Fig. 6: Mechanistic investigations. Control experiments.aReaction of1busing C6H5SO3D as the acid additive.bReaction of1b-d8using C6H5SO3H as the acid additive.cReaction of1bwithout acid additive.dIndependent-rate KIE experiments. 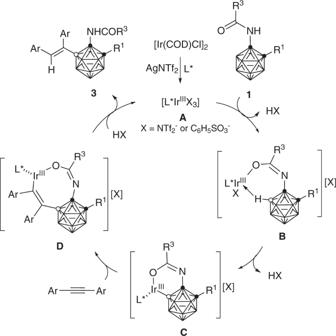Fig. 7: Proposed catalytic cycle. Possible reaction mechanism of the Ir-catalyzed enantioselective B−H alkenylation. The chiral ligand on Ir has been marked as L* for clarity. 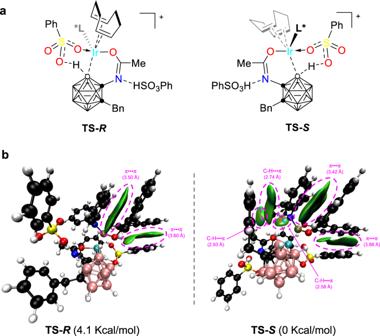Fig. 8: DFT calculated transition states. aStructures of the two transition statesTS-RandTS-Sfrom the intermediatesBtoC.bNCI analysis for the enantioselective transition statesTS-RandTS-S. Values in parentheses are distances between two interactive fragments in Å. The synthetic protocol and the characterization of compounds 1 , 3 , and 4 can be found in the Supplementary Information .